Differential regulation of the REGγ–proteasome pathway by p53/TGF-β signalling and mutant p53 in cancer cells Proteasome activity is frequently enhanced in cancer to accelerate metastasis and tumorigenesis. REGγ, a proteasome activator known to promote p53/p21/p16 degradation, is often overexpressed in cancer cells. Here we show that p53/TGF-β signalling inhibits the REGγ–20S proteasome pathway by repressing REGγ expression. Smad3 and p53 interact on the REGγ promoter via the p53RE/SBE region. Conversely, mutant p53 binds to the REGγ promoter and recruits p300. Importantly, mutant p53 prevents Smad3/N-CoR complex formation on the REGγ promoter, which enhances the activity of the REGγ–20S proteasome pathway and contributes to mutant p53 gain of function. Depletion of REGγ alters the cellular response to p53/TGF-β signalling in drug resistance, proliferation, cell cycle progression and proteasome activity. Moreover, p53 mutations show a positive correlation with REGγ expression in cancer samples. These findings suggest that targeting REGγ–20S proteasome for cancer therapy may be applicable to human tumours with abnormal p53/Smad protein status. Furthermore, this study demonstrates a link between p53/TGF-β signalling and the REGγ–20S proteasome pathway, and provides insight into the REGγ/p53 feedback loop. REGγ (also known as PA28γ, PSME3 or Ki antigen) belongs to the REG or 11S family of proteasome activator that has been shown to bind and activate 20S proteasomes [1] , [2] . REGγ activates the ubiquitin-independent degradation of steroid receptor coactivator-3 (ref. 3 ). In addition, REGγ also promotes degradation of several important regulatory proteins, including the cyclin-dependent kinase inhibitor p21 (refs 4 , 5 ). Moreover, REGγ enhances the MDM2-mediated ubiquitination and proteasomal degradation of tumour suppressor p53, inhibiting p53 accumulation and apoptosis after DNA damage [6] , [7] . Previous reports showed that REGγ-knockout mice and cells displayed reduced growth, decreased cell proliferation and increased apoptosis [8] , [9] . Growing evidence suggests that REGγ is involved in cancer progression [10] . REGγ was reported to be overexpressed in the breast [11] , thyroid [12] , colorectal [13] , lung and liver cancers [14] . However, the molecular mechanisms by which REGγ is overexpressed in multiple cancer tissues and cell lines largely remains unknown. TP53 is a sequence-specific transcription factor, which is present in a very low amount in normal cells. In response to various type of genotoxic stress, p53 is activated to regulate the expression of multiple target genes [15] , [16] . The regulation of p53-responsive genes produces proteins that interact with numerous other cellular signalling pathways, and a number of positive and negative autoregulatory feedback loops are generated [17] . The biological implications of these loops mainly depend on the function of the transcriptional targets. Yet, the p53 transcription targets and its feedback loops are not fully understood. Transforming growth factor-β (TGF-β) is a ubiquitously expressed pleiotropic cytokine that has important roles in cellular function such as apoptosis, cell cycle arrest, homeostasis, immune regulation and angiogenesis [18] , [19] . TGF-β is a potent activator of cytostatic programme in epithelial cells [20] , [21] . In the classical TGF-β pathway, ligand binding induces the assembly of type I and type II serine/threonine kinase receptors and subsequent phosphorylation of the type I receptor by constitutively active type II receptor [22] , [23] , [24] . The activated type I receptor phosphorylates cytoplasmic proteins called Smads, thus allowing the formation of heteromeric Smad complexes and their subsequent translocation to the nucleus. Once in the nucleus, these complexes control gene expression through interaction with transcription factors, coactivators and co-repressors [25] , [26] . Although TGF-β is considered a double-edged sword for its tumour suppressive and tumour-promoting functions, genetic loss of Smad function through deletion, mutation and subsequent loss of heterozygosity is a frequent event in tumours [27] . It is noteworthy that p53 is known to be required for full activity of TGF-β-mediated regulation by cooperating with Smads [28] . Inactivation of p53 has been linked to alteration of Smad-dependent TGF-β signalling [29] . Mutation of the p53 tumour suppressor gene is one of the most frequent genetic alterations in human tumours and poses a critical event in tumorigenesis, affecting tumour development, progression and responsiveness to therapy. Approximately 50% of human cancers have p53 loss-of-function mutations [30] , [31] . Mutant p53 knockin mice showed a higher frequency of tumour development and increased metastatic potential compared with p53-deficient mice [32] , [33] . Tumour-associated forms of mutant p53 can contribute to genomic instability by abrogating the mitotic spindle check point and, consequently, facilitating the generation of aneuploid cells [34] , [35] . To date, three molecular mechanisms have been described for gain of function (GOF) of mutant p53: (1) mutant p53 can bind to and inactivate the tumour suppressor proteins such as p63 and p73 (refs 36 , 37 ); (2) mutant p53 can bind to DNA and control the transcriptional regulation of putative target genes [38] , [39] ; and (3) mutant p53 can take part in the formation of large transcriptional competent complexes through which the expression of its target genes is regulated [40] , [41] . Here we report how the REGγ–20S proteasome pathway is enhanced during cancer progression. The recruitment of Smad3 and p53 at the intercalated p53RE/Smad-binding element (SBE) region in response to TGF-β provides a convergent action on REGγ expression by these tumour suppressive pathways. In addition, REGγ overexpression in diverse cancer cell lines can be specifically driven by mutant p53 that is recruited to upstream of the REGγ promoter. Moreover, mutant p53 attenuates binding of TGF-β-activated Smad3/4 complex and Nuclear receptor corepressor (N-CoR) to the SBE region of the REGγ promoter, highlighting its novel GOF ability. Silencing of REGγ alters cellular response to p53 and TGF-β signalling in drug resistance, cell proliferation, 20S proteasome activity and cell cycle progression. Our results demonstrate a role for p53/TGF-β signalling in the regulation of the REGγ–20S proteasome pathway, a new GOF for mutant p53 in enhancing the REGγ–20S proteasome pathway in cancer cells and further insight into the p53/REGγ feedback loop. TP53 represses REGγ via p53RE to generate a feedback loop In an effort to analyse transcriptional regulation of REGγ, we cloned ~2.5 Kb genomic DNA sequences upstream of the REGγ translational initiation codon. To define the transcriptional initiation site, we synthesized appropriate primers for REGγ and performed 5′-RACE (rapid amplification of complementary DNA ends) as described previously [42] . The result indicated that the REGγ transcript had a 5′-end (defined as +1) within 130 bp from the ATG site ( Supplementary Fig. S1a ). When fused to a luciferase reporter, the 2.5-Kb (−2,470/+130) and the 1.3-Kb (−1,177/+130) untranslated region (UTR) of REGγ had similar luciferase activity, whereas the (−2,470/−1,177) region produced no activity, indicating that the 1.3-Kb (−1,177/+130) UTR contains the key regulatory components for transcriptional regulation of REGγ ( Supplementary Fig. S1b ). Bioinformatic analysis, using the NCBI database, revealed that the human REGγ UTR contains four putative p53 DNA-binding sites [43] , [44] ( Fig. 1a ). A series of deletion constructs of REGγ-luc reporters were generated ( Supplementary Fig. S1c ) for measuring transcriptional activitiy. The derepression in the (−518) construct suggested a potential negative regulatory region flanking the (−738/−518) region, which correlates with the location of p53RE-2 and p53RE-3 ( Supplementary Fig. S1d ). 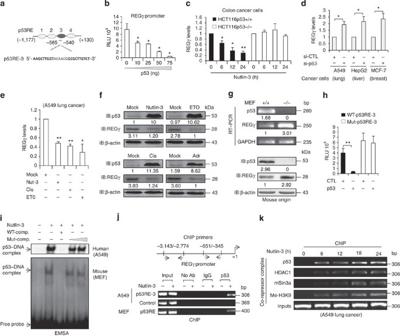Figure 1 (a) Schematic representation of putative p53-responsive elements (p53REs) with 1.3 kb region of the REGγ promoter. Dark grey colour represents critical p53RE-3. (b) H1299 cells were co-transfected with REGγ reporter construct along with an empty vector or increasing amounts of p53 for 24 h before lysis and were analysed for luciferase activity. The average was calculated based on three independent experiments. Error bars show the mean±s.d. from three technical replicates (two-tailed Student’st-test, *P<0.05). (c) HCT116 p53 (+/+) and HCT116 p53 (−/−) were treated with 10 μmol l−1Nutlin-3 for indicated time points to perform quantitative RT–PCR analysis. The average was calculated based on three independent experiments. Data are representative of three technical repeats with mean±s.d. (two-tailed Student’st-test, *P<0.05, **P<0.005). (d) A549, HepG2 and MCF-7 cells were transfected independently with siRNA specific for p53 (20 nM for 48 h) and total RNA was isolated. Data represent average of three independent experiments. Data show the mean±s.d. from three technical replicates (two-tailed Student’st-test, *P<0.05). (e,f) A549 cells were treated with different anticancer drugs such as Nutlin-3 (10 μmol l−1), Cisplatin (5 μg ml−1), ETO (10 μmol) and Adriamycin (1 μM), and were analysed by (e) RT–PCR and by (f) western blotting. (e) Error bars show the mean±s.d. from three technical replicates. (Two-tailed Student'st-test, *P<0.05, **P<0.005). (g) Comparative analysis of REGγ mRNA and protein levels in mouse embryonic fibroblast (MEF) p53 (+/+) and MEF p53 (−/−) cells. (h) H1299 cells were co-transfected with wild-type (2 μg) or mutated p53RE (2 μg) REGγ luciferase reporter constructs along with the p53 plasmid (75 ng) for 24 h and then analysed for luciferase activity. Data are representative of three independent experiments. Error bars show the mean±s.d. from three technical replicates. (two-tailed Student’st-test, **P<0.005). (i) A549 cells (upper panel) and MEF cells (lower panel) were treated with Nutlin-3 for 24 h, and EMSA assays were performed with the double-stranded oligonucleotides containing the p53RE from the REGγ promoter. (j) Schematic representation of ChIP primers. A549 cells (upper two panels) and MEF cells (lower panel) were independently treated with Nutlin-3a for 24 h, and ChIP assays were performed with anti-p53 antibody. (k) ChIP analysis of REGγ promoter in A549 cells at indicated time periods after Nutlin-3 (10 μmol l−1) treatment. Figure 1 ( a ) Schematic representation of putative p53-responsive elements (p53REs) with 1.3 kb region of the REGγ promoter. Dark grey colour represents critical p53RE-3. ( b ) H1299 cells were co-transfected with REGγ reporter construct along with an empty vector or increasing amounts of p53 for 24 h before lysis and were analysed for luciferase activity. The average was calculated based on three independent experiments. Error bars show the mean±s.d. from three technical replicates (two-tailed Student’s t -test, * P <0.05). ( c ) HCT116 p53 (+/+) and HCT116 p53 (−/−) were treated with 10 μmol l −1 Nutlin-3 for indicated time points to perform quantitative RT–PCR analysis. The average was calculated based on three independent experiments. Data are representative of three technical repeats with mean±s.d. (two-tailed Student’s t -test, * P <0.05, ** P <0.005). ( d ) A549, HepG2 and MCF-7 cells were transfected independently with siRNA specific for p53 (20 nM for 48 h) and total RNA was isolated. Data represent average of three independent experiments. Data show the mean±s.d. from three technical replicates (two-tailed Student’s t -test, * P <0.05). ( e , f ) A549 cells were treated with different anticancer drugs such as Nutlin-3 (10 μmol l −1 ), Cisplatin (5 μg ml −1 ), ETO (10 μmol) and Adriamycin (1 μM), and were analysed by ( e ) RT–PCR and by ( f ) western blotting. ( e ) Error bars show the mean±s.d. from three technical replicates. (Two-tailed Student's t -test, * P <0.05, ** P <0.005). ( g ) Comparative analysis of REGγ mRNA and protein levels in mouse embryonic fibroblast (MEF) p53 (+/+) and MEF p53 (−/−) cells. ( h ) H1299 cells were co-transfected with wild-type (2 μg) or mutated p53RE (2 μg) REGγ luciferase reporter constructs along with the p53 plasmid (75 ng) for 24 h and then analysed for luciferase activity. Data are representative of three independent experiments. Error bars show the mean±s.d. from three technical replicates. (two-tailed Student’s t -test, ** P <0.005). ( i ) A549 cells (upper panel) and MEF cells (lower panel) were treated with Nutlin-3 for 24 h, and EMSA assays were performed with the double-stranded oligonucleotides containing the p53RE from the REGγ promoter. ( j ) Schematic representation of ChIP primers. A549 cells (upper two panels) and MEF cells (lower panel) were independently treated with Nutlin-3a for 24 h, and ChIP assays were performed with anti-p53 antibody. ( k ) ChIP analysis of REGγ promoter in A549 cells at indicated time periods after Nutlin-3 (10 μmol l −1 ) treatment. Full size image To investigate whether p53 transcriptionally regulates REGγ, we co-transfected the REGγ-luc reporter into H1299 cells. Repression was observed when the reporter construct was co-transfected with different doses of p53 ( Fig. 1b ). Derepression of REGγ also occurred in p53-depleted HCT116 cells ( Supplementary Fig. S2a ). In response to Nutlin-3, inhibition of the REGγ transcript was detected in HCT116 (p53+/+) but not in the isogenic HCT116 (p53−/−) cells ( Fig. 1c and Supplementary Fig. S2b ). Silencing p53 by short interfering RNA (siRNA) in multiple cancer cells greatly increased REGγ mRNA levels compared with controls ( Fig. 1d and Supplementary Fig. S2c ). Similar to Nutlin-3, cisplatin and etoposide (ETO) also significantly reduced both REGγ mRNA and protein expressions ( Fig. 1e,f ). Likewise, upregulation of REGγ was also observed in p53−/− mouse embryonic fibroblast cells ( Fig. 1g ). Next, we attempted to identify the regulatory region conferring p53 responsiveness within the REGγ promoter. Interestingly, only p53RE-3 displayed strong binding to p53 by electrophoretic mobility shift assay (EMSA; Supplementary Fig. S2d ). Mutation of the p53RE-3 construct abolished its response to p53 inhibition, validating that p53 binds to p53RE-3 to repress REGγ transcription ( Fig. 1h ). We further confirmed p53 binding to p53RE-3 by EMSA assay, which resulted in the formation of a p53–DNA complex ( Fig. 1i , upper panel). We obtained similar results for the p53RE-3 probe using recombinant p53 protein ( Supplementary Fig. S2e ). Intriguingly, EMSA analysis also revealed p53 binding to a probe derived from mouse REGγ UTR ( Fig. 1i , lower panel). To determine whether p53 directly binds to p53RE in vivo , a chromatin immunoprecipitation (ChIP) assay was performed using the primers derived from the REGγ promoter ( Fig. 1j ). The anti-p53 antibody specifically pulled down DNA fragments corresponding to the p53RE-3 region ( Fig. 1j , upper two panels and Supplementary Fig. S2f ). Moreover, the ChIP assay also suggested p53 binding to p53RE in the UTR of mouse REGγ using mouse embryonic fibroblast cells treated with Nutlin-3 ( Fig. 1j , lower panel). It was previously reported that p53 has been associated with the recruitment of histone deacetylase to repress its target genes [45] . Thus, the ChIP assays also demonstrated a time-course-dependent recruitment of p53 and mSIN3A-HDAC1 co-repressor complex to the REGγ promoter ( Fig. 1k ). Importantly, this co-repressor complex was preferentially associated with a repressive chromatin status in the REGγ promoter, as indicated from the enrichment of Me-H3K9 ( Fig. 1k ), a marker of repressed chromatin [46] . Taken together, these data demonstrate that p53 directly binds to the UTR of both human and mouse REGγ genes to mediate mSIN3A/HDAC1-dependent transrepression. Given that REGγ negatively regulates p53 protein levels, our findings provide a new mechanism for feedback regulation between p53 and REGγ pathway in cancer cells. TGF-β inhibits the REGγ–proteasome pathway via Smad complex As Smad3 and Smad4 specifically recognize the DNA sequence AGAC or GTCT [47] , the presence of multiple SBE in the REGγ promoter prompted us to analyse the potential of TGF-β in regulating REGγ. In a dose-dependent manner, TGF-β was able to repress the transcriptional activity of the REGγ-luc reporter ( Fig. 2a ). Ectopic expression of Smad3/4 combination strongly inhibited REGγ activity in comparison with Smad2/4 combination ( Fig. 2b ). Furthermore, expression of REGγ mRNA was also inhibited in response to TGF-β ( Fig. 2c , and Supplementary Fig. S3a,b ). TGF-β was unable to repress REGγ in Smad3 knockdown cells ( Fig. 2d ). TGF-β treatment also decreased the REGγ protein level in multiple cancer cell lines ( Fig. 2e ). Similarly, depletion of Smad3 in cancer cells led to the elevated expression of REGγ ( Fig. 2f ). 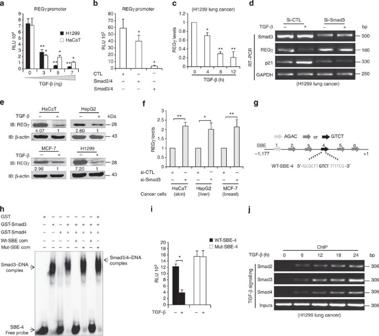Figure 2: Smad complex represses the REGγ–proteasome pathway through SBE. (a) H1299 and HaCaT cells were transfected independently with REGγ reporter construct (2 μg), treated with different doses of TGF-β for 24 h before lysis and were analysed for luciferase activity. Data are representative of three technical repeats with mean±s.d. (two-tailed Student’st-test, *P<0.05, **P<0.005). (b) H1299 cells were co-transfected with REGγ reporter construct (2 μg) in combination with either Smad2/4 (100 ng) or Smad3/4 (100 ng) expression plasmids for 24 h and then analysed for luciferase activity. Data are representative of three technical repeats with mean±s.d. (two-tailed Student’st-test, *P<0.05). (c) H1299 were incubated in the absence or presence of 5 ng ml−1TGF-β for indicated time points. Total RNA was isolated and subjected to quantitative RT–PCR. Data are representative of three technical replicates with mean±s.d. (two-tailed Student’st-test, *P<0.05, **P<0.005). (d) H1299 cells were transfected with siRNA directed against Smad3 (20 nM). After 48 h of transfection, cells were treated with 5 ng ml−1TGF-β for 12 h and semiquantitative RT–PCR was performed to analyse REGγ, Smad3 and p21 mRNA levels. (e) HaCaT, HepG2, MCF-7 and H1299 cells were treated with 5 ng ml−1TGF-β and analysed by western blotting. (f) HaCaT, HepG2 and MCF-7 cells were transfected independently with siRNA specific for Smad3 (20 nM, for 48 h) and total RNA was isolated. Error bars show the mean±s.d. from three technical replicates (two-tailed Student’st-test, *P<0.05, **P<0.005). (g) Schematic representation of putative SBE boxes in the REGγ promoter. The black arrows indicate the functional SBE in the REGγ promoter. (h) EMSA assay was performed using purified glutathioneS-transferase (GST)-Smad3 protein. Fifty nanograms of GST-Smad3 protein were incubated with32P-radiolabelled probe containing SBE box from the REGγ promoter. (i) H1299 cells were transfected with wild-type (2 μg) or mutated (2 μg) SBE REGγ luciferase reporter constructs. Cells were then left untreated or treated with 5 ng ml−1TGF-β for 24 h and luciferase activity was measured. Error bars show the mean±s.d. from three technical replicates. Data are representative of three independent experiments (two-tailed Student’st-test, *P<0.05). (j) H1299 cells were treated with 5 ng ml−1TGF-β for indicated time and ChIP analyses were performed with indicated antibodies. Figure 2: Smad complex represses the REGγ–proteasome pathway through SBE. ( a ) H1299 and HaCaT cells were transfected independently with REGγ reporter construct (2 μg), treated with different doses of TGF-β for 24 h before lysis and were analysed for luciferase activity. Data are representative of three technical repeats with mean±s.d. (two-tailed Student’s t -test, * P <0.05, ** P <0.005). ( b ) H1299 cells were co-transfected with REGγ reporter construct (2 μg) in combination with either Smad2/4 (100 ng) or Smad3/4 (100 ng) expression plasmids for 24 h and then analysed for luciferase activity. Data are representative of three technical repeats with mean±s.d. (two-tailed Student’s t -test, * P <0.05). ( c ) H1299 were incubated in the absence or presence of 5 ng ml −1 TGF-β for indicated time points. Total RNA was isolated and subjected to quantitative RT–PCR. Data are representative of three technical replicates with mean±s.d. (two-tailed Student’s t -test, * P <0.05, ** P <0.005). ( d ) H1299 cells were transfected with siRNA directed against Smad3 (20 nM). After 48 h of transfection, cells were treated with 5 ng ml −1 TGF-β for 12 h and semiquantitative RT–PCR was performed to analyse REGγ, Smad3 and p21 mRNA levels. ( e ) HaCaT, HepG2, MCF-7 and H1299 cells were treated with 5 ng ml −1 TGF-β and analysed by western blotting. ( f ) HaCaT, HepG2 and MCF-7 cells were transfected independently with siRNA specific for Smad3 (20 nM, for 48 h) and total RNA was isolated. Error bars show the mean±s.d. from three technical replicates (two-tailed Student’s t -test, * P <0.05, ** P <0.005). ( g ) Schematic representation of putative SBE boxes in the REGγ promoter. The black arrows indicate the functional SBE in the REGγ promoter. ( h ) EMSA assay was performed using purified glutathione S -transferase (GST)-Smad3 protein. Fifty nanograms of GST-Smad3 protein were incubated with 32 P-radiolabelled probe containing SBE box from the REGγ promoter. ( i ) H1299 cells were transfected with wild-type (2 μg) or mutated (2 μg) SBE REGγ luciferase reporter constructs. Cells were then left untreated or treated with 5 ng ml −1 TGF-β for 24 h and luciferase activity was measured. Error bars show the mean±s.d. from three technical replicates. Data are representative of three independent experiments (two-tailed Student’s t -test, * P <0.05). ( j ) H1299 cells were treated with 5 ng ml −1 TGF-β for indicated time and ChIP analyses were performed with indicated antibodies. Full size image Next, we sought to define potentially functional SBE in the REGγ promoter. We designed oligo probes containing each of the putative SBE, respectively ( Fig. 2g ), and found that only SBE-4, but not other SBEs, could have strongly bound to Smad3 ( Supplementary Fig. S3c ). Furthermore, formation of the DNA–Smad3/4 complex was observed on SBE-4 (Fig. 2h ). We also observed the binding of cellular Smads to SBE-4 in response to TGF-β ( Supplementary Fig. S3d ). Moreover, mutation of SBE-4 within the 1.3-Kb REGγ-luc reporter blunted its response to TGF-β inhibition, further validating that an activated Smad complex binds to SBE-4 to repress REGγ transcription ( Fig. 2i ). Finally, we detected recruitment of Smad2/3 and Smad4 to the TGF-β responsive region (−796/−481; Supplementary Fig. S3e,f). Recruitment of Smad proteins to the REGγ promoter occurred within 6 h of TGF-β addition and accumulated with increased time of TGF-β treatment ( Fig. 2j ). In conclusion, the Smad signalling pathway is required for REGγ repression in response to TGF-β, suggesting a potential mechanism by which loss of Smad3 in diverse cancer cells may result in an elevated expression of REGγ. Thus, Smad proteins serve as key transcriptional regulators for the REGγ–proteasome pathway to maintain low expression of REGγ in cancer cells. p53 and Smad3 interacts via p53RE/SBE in response to TGF-β Under normal phenotypic conditions, both TGF-β and activated p53 act as gene-specific transcription factors regulating multiple transcriptional targets to achieve tumour suppressive effects [48] . The p53 protein has been identified as a gene-specific partner for Smads and is important for the formation and stabilization of Smad–DNA complexes. Smad2 and Smad3, but not Smad4, directly interact with p53 (ref. 28 ). Thus, Smad2/3, bound to TGF-β-responsive element(s), may bridge p53, bound at the p53-binding element, with the Smad complex, allowing additive or synergistic activation of transcription [28] , [49] . These hints prompted us to search for intercalated p53RE/SBE site on the REGγ promoter. Intriguingly, we found a p53RE/SBE regulatory region between (−565/−540) in the REGγ promoter, which comprises overlapping p53RE-3/SBE-4 ( Fig. 3a ). Expression of either p53 or Smad3/4 with the p53RE/SBE-luc construct repressed reporter activities, whereas these repressions were more dramatic in the presence of TGF-β ( Fig. 3b ). Strikingly, coexpression of p53 and Smad3/4 along with TGF-β was significantly more efficient than either p53 or Smad3/4 alone in their regulatory actions ( Fig. 3b ). We also obtained similar results for (TA-p63+Smad3/4) and (TA-p73+Smad3/4) combinations ( Supplementary Fig. S4a,b ). We next verified repression of the REGγ gene in A549 cells treated with TGF-β or Nutlin-3, alone or in combination. Either TGF-β or Nutlin-3 can elicit overt inhibition of REGγ mRNA levels, whereas this reduction was much more significant when cells were treated with the TGF-β/Nutlin-3 combination ( Fig. 3c,d ). Moreover, cosilencing of p53/Smad3 resulted in more than twofold upregulation of REGγ expression ( Fig. 3e ), indicating that p53 and Smad3/4 act as transcriptional co-repressors on the REGγ promoter. 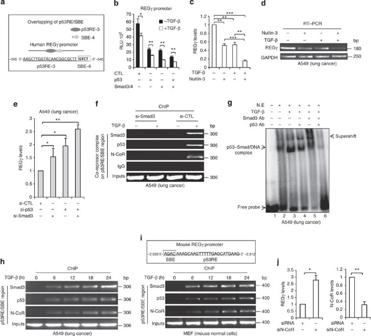Figure 3: TGF-β stimulates the formation of p53/Smad3/N-CoR on REGγ promoter via p53RE/SBE site. (a) Schematic representation of p53RE/SBE overlapping region on REGγ promoter. (b) H1299 cells were co-transfected with expression vectors encoding p53/Smad3/4, both alone and in combination, left untreated or treated with 5 ng ml−1TGF-β for 24 h before lyses and were analysed for luciferase activity. Error bars show the mean±s.d. from three technical replicates. Data are representative of three independent experiments (two-tailed Student’st-test, *P<0.05, **P<0.005). (c,d) A549 cells were treated with 5 ng ml−1TGF-β and 10 μmol l−1Nutlin-3 either alone or in combination for 24 h and RT–PCR analysis was performed. Error bars show the mean±s.d. from three technical replicates (two-tailed Student’st-test, **P<0.005, ***P<0.0005). (e) A549 cells were transfected with siRNA directed against Smad3 (20 nM) or p53 (20 nM), either alone or in combination for 48 h. Total RNA was extracted for quantitative RT–PCR to analyse REGγ mRNA level. Data are representative of three technical repeats with mean±s.d. (two-tailed Student’st-test, *P<0.05, **P<0.005). (f) ChIP analysis indicating that knockdown of Smad3 prevents the recruitment of Smad3, p53 and N-CoR to the REGγ promoter in response to TGF-β in A549 cell lines. (g) A549 cells were treated with 5 ng ml−1TGF-β for 24 h and nuclear extracts were subjected to EMSA analysis with32P-end-labelled probes corresponding to the p53RE/SBE region from the REGγ promoter. Antibodies against Smad3 and p53 were added as indicated. (h) TGF-β enhances Smad3/p53/N-CoR recruitment at the p53RE/SBE on human REGγ promoter. (h) A549 cells were treated with 5 ng ml−1TGF-β for the indicated time and ChIP analyses were performed with the antibodies specific for Smad3, p53 and N-CoR. (i) Schematic representation of p53RE/SBE site on mouse REGγ promoter (upper panel) and showing the recruitment of Smad3, p53 and N-CoR in mouse mouse embryonic fibroblast (MEF) cell lines in response to TGF-β (lower panel). (j) A549 cells were treated with (20 nM) N-CoR siRNA for 48 h and were analysed by RT–PCR (left panel). Knockdown efficiency of N-CoR in A549 cells (right panel). Error bars show the mean±s.d. from three technical replicates (two-tailed Student’st-test, *P<0.05, **P<0.005). Figure 3: TGF-β stimulates the formation of p53/Smad3/N-CoR on REGγ promoter via p53RE/SBE site. ( a ) Schematic representation of p53RE/SBE overlapping region on REGγ promoter. ( b ) H1299 cells were co-transfected with expression vectors encoding p53/Smad3/4, both alone and in combination, left untreated or treated with 5 ng ml −1 TGF-β for 24 h before lyses and were analysed for luciferase activity. Error bars show the mean±s.d. from three technical replicates. Data are representative of three independent experiments (two-tailed Student’s t -test, * P <0.05, ** P <0.005). ( c , d ) A549 cells were treated with 5 ng ml −1 TGF-β and 10 μmol l −1 Nutlin-3 either alone or in combination for 24 h and RT–PCR analysis was performed. Error bars show the mean±s.d. from three technical replicates (two-tailed Student’s t -test, ** P <0.005, *** P <0.0005). ( e ) A549 cells were transfected with siRNA directed against Smad3 (20 nM) or p53 (20 nM), either alone or in combination for 48 h. Total RNA was extracted for quantitative RT–PCR to analyse REGγ mRNA level. Data are representative of three technical repeats with mean±s.d. (two-tailed Student’s t -test, * P <0.05, ** P <0.005). ( f ) ChIP analysis indicating that knockdown of Smad3 prevents the recruitment of Smad3, p53 and N-CoR to the REGγ promoter in response to TGF-β in A549 cell lines. ( g ) A549 cells were treated with 5 ng ml −1 TGF-β for 24 h and nuclear extracts were subjected to EMSA analysis with 32 P-end-labelled probes corresponding to the p53RE/SBE region from the REGγ promoter. Antibodies against Smad3 and p53 were added as indicated. ( h ) TGF-β enhances Smad3/p53/N-CoR recruitment at the p53RE/SBE on human REGγ promoter. ( h ) A549 cells were treated with 5 ng ml −1 TGF-β for the indicated time and ChIP analyses were performed with the antibodies specific for Smad3, p53 and N-CoR. ( i ) Schematic representation of p53RE/SBE site on mouse REGγ promoter (upper panel) and showing the recruitment of Smad3, p53 and N-CoR in mouse mouse embryonic fibroblast (MEF) cell lines in response to TGF-β (lower panel). ( j ) A549 cells were treated with (20 nM) N-CoR siRNA for 48 h and were analysed by RT–PCR (left panel). Knockdown efficiency of N-CoR in A549 cells (right panel). Error bars show the mean±s.d. from three technical replicates (two-tailed Student’s t -test, * P <0.05, ** P <0.005). Full size image Next, we aimed to address the molecular details of the potential interaction of p53 and Smad proteins at the p53RE-3/SBE-4 region. We silenced Smad3 expression in the A549 cell to determine whether recruitment of p53 to REGγ promoter depends on Smad3 in response to TGF-β. ChIP analysis showed no recruitment of Smad3, p53 and N-CoR in Smad3-depleted cells in the presence of TGF-β, which was comparable with control cell lines, suggesting that activated Smad3 interacts with p53 at the p53RE-3/SBE-4 region in response to TGF-β, and entails recruitment of p53 to the REGγ promoter ( Fig. 3f ). To define binding of these proteins to p53RE-3/SBE-4 regulatory region, we performed an EMSA assay. Incubation of nuclear extracts with a 26-nt probe resulted in formation of a putative p53–Smad–DNA complex, which is enhanced in the presence of TGF-β ( Fig. 3g , lanes 2 and 3). Addition of both antibodies against p53 and Smad3 nearly abolished all bands ( Fig. 3g , lane 6), indicating that these complexes contained both p53 and Smad3 proteins. Consistent with our in vitro protein–DNA interaction analysis, ChIP assays revealed that TGF-β stimulated corecruitment of Smad3/p53/N-CoR to this region, suggesting the cooperation between p53 and Smads to further repress REGγ ( Fig. 3h ). Intriguingly, sequence analysis of the mouse REGγ promoter also showed p53RE/SBE site between the (−2,939/−2,912) region ( Fig. 3i ). ChIP assay disclosed binding of Smad3/p53/N-CoR to this region as well ( Fig. 3i ). Next, we depleted expression of N-CoR using specific siRNA to validate the biological impact of N-CoR on REGγ regulation. Reverse transcriptase–PCR (RT–PCR) analysis revealed that the REGγ mRNA level was elevated in N-CoR knockdown cells ( Fig. 3j ). Taken together, our data suggest that synergism/collaboration between p53 and TGF-β occurs on the REGγ promoter through the p53RE/SBE region, which contributes to further inhibition of the REGγ–proteasome activity. Importantly, our data suggest crosstalk between these two key pathways, not only in human cancer cell lines but also in non-cancer mouse cells. Mutant p53 interacts and recruits p300 to induce REGγ Mutant p53 was previously detected on the promoters of some target genes, including CD95 (ref. 50 ), EGR1 (ref. 51 ), MSP-1 (ref. 52 ), GRO-1 (ref. 53 ), ID2 (ref. 54 ) and ID4 (ref. 55 ), and this was observed in the absence of external stimuli, implying that mutant p53 can directly bind to and regulate its target genes. To understand whether mutant p53 regulate REGγ, we co-transfected the REGγ-luc reporter with increasing amounts of mutant p53-R175H and observed the dose-dependent transactivation of the REGγ-luciferase reporter ( Fig. 4a ). Consistently, expressing REGγ-luc reporter construct in UMSCC-1 cell lines stably expressing an empty vector, p53 or p53-R175H also suggested a role for mutant p53 to promote REGγ transcription ( Supplementary Fig. S5a ). Moreover, all coexpressed constructs containing hotspot p53 mutations significantly activated transcription of REGγ reporter in the H1299 cell ( Fig. 4b ). To investigate the impact of endogenous mutant p53 on REGγ expression, we silenced mutant p53 in multiple cancer cells. Depletion of mutant p53 in these cells reduced the level of REGγ transcripts and proteins ( Fig. 4c,d , and Supplementary Fig. S5b,c ). Conversely, H1299 cells stably expressing p53-R175H strongly induced REGγ protein levels compared with control cells ( Fig. 4e , left panel). Strikingly, immortalized oral cancer cells from mice with p53 mutation at amino acids 172 (R172H) [56] displayed significant upregulation in REGγ protein level compared with p53−/− oral cancer cells ( Fig. 4e , right panel). 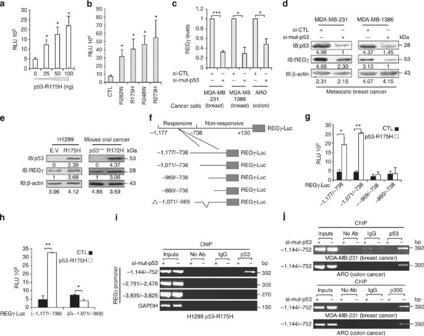Figure 4: Mutant p53 enhances REGγ expression via p300 recruitment. (a) H1299 cells were co-transfected with the REGγ reporter construct (2 μg) along with empty vector or increasing amounts of p53-R175H for 24 h before lysis and were analysed for luciferase activity. Data are representative of three technical replicates with mean±s.d. (two-tailed Student’st-test, *P<0.05). (b) H1299 cells were co-transfected with REGγ promoter (2 μg) in combination with different mutant p53 proteins such as p53-R282W (50 ng), p53-R175H (50 ng), p53-R248W (50 ng) and p53-R273H (50 ng) for 24 h before lysis and were analysed for luciferase activity. Error bars show the mean±s.d. from three technical replicates (two-tailed Student’st-test, *P<0.05). (c) MDA-MB-231, MDA-MB-1386 and ARO cells were transfected with the siRNA specific for p53 (20 nM), and after 48 h, total RNA was subjected to quantitative RT–PCR analysis. Error bars show the mean±s.d. from three technical replicates (two-tailed Student’st-test, *P<0.05, ***P<0.0005). (d) MDA-MB-231 and MDA-MB-1386 cells were transfected with siRNA directed against p53 (20 nM) for 72 h and were analysed by western blotting. (e) H1299 cells stably expressing either empty vector (E.V) or p53-R175H, and immortalized oral cancer cells from p53 (−/−) or p53-R172H mice were subjected to western blot analysis (right panel). (f) Schematic representation of different deletion constructs of REGγ promoter. (g) Full-length (−1,177/−738) and different truncated constructs of REGγ within this region (each 2 μg) were co-transfected in H1299 cells along with p53-R175H (100 ng) for 24 h before lyses were and then analysed for luciferase activity. Error bars show the mean±s.d. from three technical replicates (two-tailed Student’st-test, *P<0.05, **P<0.005). (h) Deletion of (−1,071/−969) region abolishes the transactivation of REGγ by mutant p53. Error bars show the mean±s.d. from three technical replicates (two-tailed Student’st-test, *P<0.05, **P<0.005). (i) Binding of mutant p53 to the REGγ promoter in H1299 p53-R175H was measured by ChIP analysis. (j) Binding of endogenous mutant p53 to the REGγ promoter in MDA-MB-231 and ARO cells were measured by ChIP analysis (upper two panels) and recruitment of p300 to REGγ promoter by ChIP analysis (lower two panels). Figure 4: Mutant p53 enhances REGγ expression via p300 recruitment. ( a ) H1299 cells were co-transfected with the REGγ reporter construct (2 μg) along with empty vector or increasing amounts of p53-R175H for 24 h before lysis and were analysed for luciferase activity. Data are representative of three technical replicates with mean±s.d. (two-tailed Student’s t -test, * P <0.05). ( b ) H1299 cells were co-transfected with REGγ promoter (2 μg) in combination with different mutant p53 proteins such as p53-R282W (50 ng), p53-R175H (50 ng), p53-R248W (50 ng) and p53-R273H (50 ng) for 24 h before lysis and were analysed for luciferase activity. Error bars show the mean±s.d. from three technical replicates (two-tailed Student’s t -test, * P <0.05). ( c ) MDA-MB-231, MDA-MB-1386 and ARO cells were transfected with the siRNA specific for p53 (20 nM), and after 48 h, total RNA was subjected to quantitative RT–PCR analysis. Error bars show the mean±s.d. from three technical replicates (two-tailed Student’s t -test, * P <0.05, *** P <0.0005). ( d ) MDA-MB-231 and MDA-MB-1386 cells were transfected with siRNA directed against p53 (20 nM) for 72 h and were analysed by western blotting. ( e ) H1299 cells stably expressing either empty vector (E.V) or p53-R175H, and immortalized oral cancer cells from p53 (−/−) or p53-R172H mice were subjected to western blot analysis (right panel). ( f ) Schematic representation of different deletion constructs of REGγ promoter. ( g ) Full-length (−1,177/−738) and different truncated constructs of REGγ within this region (each 2 μg) were co-transfected in H1299 cells along with p53-R175H (100 ng) for 24 h before lyses were and then analysed for luciferase activity. Error bars show the mean±s.d. from three technical replicates (two-tailed Student’s t -test, * P <0.05, ** P <0.005). ( h ) Deletion of (−1,071/−969) region abolishes the transactivation of REGγ by mutant p53. Error bars show the mean±s.d. from three technical replicates (two-tailed Student’s t -test, * P <0.05, ** P <0.005). ( i ) Binding of mutant p53 to the REGγ promoter in H1299 p53-R175H was measured by ChIP analysis. ( j ) Binding of endogenous mutant p53 to the REGγ promoter in MDA-MB-231 and ARO cells were measured by ChIP analysis (upper two panels) and recruitment of p300 to REGγ promoter by ChIP analysis (lower two panels). Full size image Next, reporter assays were performed with various truncated REGγ-luc constructs to determine the region responsive to mutant p53. The 1.39Kb REGγ-luc reporter construct (−1,177/+130) was responsive to mutant p53 transactivation, whereas a truncated REGγ-luc construct (−738/+130) remained unresponsive to mutant p53 ( Supplementary Fig. S5d ), indicating a cis -element within the (−1,177/−738) region for mutant p53. To further define the mutant p53-responsive region in the REGγ UTR, we generated different REGγ-Luc deletion constructs ( Fig. 4f ) and found that the region between (−1,071/−969) is essential for mutant p53-dependent transcription ( Fig. 4g ). Deletion of this region (−1,071/−969) abolished the capability of mutant p53 to transactivate the REGγ promoter ( Fig. 4h ), indicating that sequence from (−1,071/−969) may be required for mutant p53 binding. ChIP assays were carried out to examine the association of endogenous mutant p53 with this regulatory region. Following immunoprecipitation of chromatin from H1299 p53-R175H stable cell lines transfected with either sip53 or control siRNA, we observed recruitment of mutant p53 to a region flanking (−1,144/−752) in the REGγ UTR, but not in regions 2 kb further upstream or in cells having depleted mutant p53 ( Fig. 4i ). We also examined REGγ promoter occupancy by naturally occurring mutant p53 with ChIP analysis in human breast cancer and colon cancers cell lines. We detected recruitment of mutant p53 (p53-R280K and p53-R273H) to REGγ promoters in MDA-MB-231 and ARO cells ( Fig. 4j , upper two panels). Interestingly, ChIP analysis also revealed that p300 bound to the REGγ promoter in mutant p53 (MDA-MB-231 and ARO)-containing cells but not to cells with depleted mutant p53 ( Fig. 4j , lower two panels). Altogether, our results demonstrate that the REGγ–20S proteasome pathway is likely to be a common target for different mutant p53 proteins in multiple human cancer cells and mouse oral cancer cells. Moreover, induction of REGγ occurs through recruitment of mutant p53 proteins along with p300 onto the specific regulatory region in REGγ UTR. These findings disclose a new regulatory venue for mutant p53-mediated expression of proteasome activator REGγ in different cancer cell types. Mutant p53 prevents Smad3/N-CoR formation on REGγ promoter A previous study showed that mutant p53 attenuates the TGF-β pathway by repressing the TGF-βRII gene, delaying or reducing phosphorylation of Smad2 by TGF-βRI [57] . Because of the negative and positive responses of REGγ promoter to TGF-β and mutant p53, respectively, we investigated the effect of TGF-β/Smad3/4 signalling on REGγ expression in mutant p53-expressing cells. We transfected p53-null H1299 cells with Smad3/4 and p53-R175H expression plasmids independently or in combination, and found that mutant p53 was able to attenuate the Smad3/4-mediated inhibition of REGγ promoter in fold changes ( Fig. 5a ). Furthermore, we also observed a significant reduction in REGγ mRNA and protein levels in H1299 control cells when stimulated with TGF-β, whereas this TGF-β-mediated inhibition was alleviated in cells harbouring p53-R175H ( Fig. 5b,c ). We obtained similar results in naturally harbouring mutant p53 MDA-MB-231 (p53-R280K) and MDA-MB-1386 (p53-R282W) cells by comparing cells with or without mutant p53 silencing ( Fig. 5d,e ). These results prompted us to test the influence of mutant p53 protein on binding of TGF-β-activated Smad3/4 complex to the REGγ promoter. For comparison, H1299 cells were infected with a control viral vector, or vectors encoding p53 or p53-R175H, followed by ChIP analysis. We detected the recruitment of Smad3 to REGγ promoter in the presence of TGF-β in control and p53-expressing cells ( Fig. 5f ). Conversely, we observed little binding of Smad3 in p53-R175H-expressing H1299 cells ( Fig. 5f , upper panel). We also validated these observations by ChIP assays in UMSCC-1 cells, stably integrated with an empty vector, p53 or hotspot p53-R175H mutant allele ( Fig. 5f , lower panel). We obtained similar results in naturally occurring mutant p53 MDA-MB-231 ( Fig. 5g ) and stably expressing mutant p53 H1299 cell lines ( Fig. 5h ), respectively. 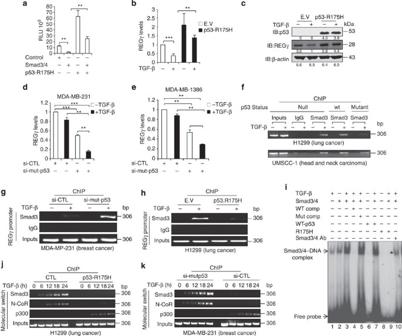Figure 5: Mutant p53 antagonizes recruitment of the Smad3/N-CoR complex on the REGγ promoter. (a) H1299 were co-transfected with Smad3/4 and p53-R175H expression plasmids independently or in combination and were analysed for luciferase activity. Data are representative of three technical repeats with mean±s.d. (two-tailed Student’st-test, **P<0.005). (b,c) H1299 cells stably expressing either p53-R175H mutant or empty vectors (E.V) were left untreated or treated with 5 ng ml−1TGF-β and were analysed by RT–PCR and western blotting, respectively. Data are representative of three technical repeats with mean±s.d. (two-tailed Student’st-test, **P<0.005, ***P<0.0005). (d,e) MDA-MB-231 and MDA-MB-1386 cells were left non-transfected (−) or transfected (+) with siRNA (20 nM) against mutant p53, and then stimulated with TGF-β and analysed by quantitative RT–PCR. Data are representative of three technical repeats with mean±s.d. (two-tailed Student’st-test, **P<0.005, ***P<0.0005). (f) H1299 cells were infected either with an E.V, p53 or p53-R175H encoding vectors, and left untreated or treated with 5 ng ml−1TGF-β for 24 h (upper panel). UMSSC-1 cells stably expressing an empty vector, p53 or p53-R175H vectors were treated similar to those in the upper panel (lower panel). ChIP analysis was performed with antibodies recognizing Smad3. (g) MDA-MB-231 cells expressing endogenous mutant p53 and (h) H1299 cells stably expressing p53-R175H were incubated in the presence or absence of 5 ng ml−1TGF-β for 24 h and ChIP analyses were performed. (i) H1299 cells were transfected with Smad3/4, p53 or p53-R175H expression plasmids alone or in combination of (Smad3/4 and p53) and (Smad3/4 and p53-R175H), and then stimulated with 5 ng ml−1TGF-β for 24 h. Nuclear extracts were prepared and subjected to EMSA analysis with32P-end-labelled probes corresponding to cognate SBE box from the REGγ promoter. *Blocking of Smad3/4 complex formation by mutant p53-R175H. (j,k) Mutant p53 reverts TGF-β induced repression of theREGγgene through p300. (j) H1299 cells expressing either E.V or p53-R175H, and (k) MDA-MB-231 cells were stimulated with 5 ng ml−1TGF-β for indicated time points, and subjected to ChIP analysis with indicated antibodies. Figure 5: Mutant p53 antagonizes recruitment of the Smad3/N-CoR complex on the REGγ promoter. ( a ) H1299 were co-transfected with Smad3/4 and p53-R175H expression plasmids independently or in combination and were analysed for luciferase activity. Data are representative of three technical repeats with mean±s.d. (two-tailed Student’s t -test, ** P <0.005). ( b , c ) H1299 cells stably expressing either p53-R175H mutant or empty vectors (E.V) were left untreated or treated with 5 ng ml −1 TGF-β and were analysed by RT–PCR and western blotting, respectively. Data are representative of three technical repeats with mean±s.d. (two-tailed Student’s t -test, ** P <0.005, *** P <0.0005). ( d , e ) MDA-MB-231 and MDA-MB-1386 cells were left non-transfected (−) or transfected (+) with siRNA (20 nM) against mutant p53, and then stimulated with TGF-β and analysed by quantitative RT–PCR. Data are representative of three technical repeats with mean±s.d. (two-tailed Student’s t -test, ** P <0.005, *** P <0.0005). ( f ) H1299 cells were infected either with an E.V, p53 or p53-R175H encoding vectors, and left untreated or treated with 5 ng ml −1 TGF-β for 24 h (upper panel). UMSSC-1 cells stably expressing an empty vector, p53 or p53-R175H vectors were treated similar to those in the upper panel (lower panel). ChIP analysis was performed with antibodies recognizing Smad3. ( g ) MDA-MB-231 cells expressing endogenous mutant p53 and ( h ) H1299 cells stably expressing p53-R175H were incubated in the presence or absence of 5 ng ml −1 TGF-β for 24 h and ChIP analyses were performed. ( i ) H1299 cells were transfected with Smad3/4, p53 or p53-R175H expression plasmids alone or in combination of (Smad3/4 and p53) and (Smad3/4 and p53-R175H), and then stimulated with 5 ng ml −1 TGF-β for 24 h. Nuclear extracts were prepared and subjected to EMSA analysis with 32 P-end-labelled probes corresponding to cognate SBE box from the REGγ promoter. *Blocking of Smad3/4 complex formation by mutant p53-R175H. ( j , k ) Mutant p53 reverts TGF-β induced repression of the REGγ gene through p300. ( j ) H1299 cells expressing either E.V or p53-R175H, and ( k ) MDA-MB-231 cells were stimulated with 5 ng ml −1 TGF-β for indicated time points, and subjected to ChIP analysis with indicated antibodies. Full size image In addition, we examined the effect of mutant p53 on Smad3/4-binding affinity to corresponding SBE-4 on the REGγ promoter. Nuclear extracts were prepared from H1299 cells co-transfected with Smad3/4, p53 and p53-R175H expression plasmids, alone or in combination (Smad3/4+p53 or Smad3/4+p53-R175H), followed by TGF-β treatment. We believe the EMSA assay probe containing SBE-4 displayed formation of a Smad3/4–DNA complex, as this complex was strongly enhanced after TGF-β stimulation and attenuated after the addition of Smad antibodies ( Fig. 5i , lanes 3 and 10). Strikingly, the binding capacity of this Smad3/4 complex to the corresponding SBE-4 oligo was completely abolished by mutant p53-R175H ( Fig. 5i , lane 9), suggesting that mutant p53 proteins antagonize TGF-β signalling by inhibiting the binding of Smad complexes to regulatory elements on REGγ promoter. Moreover, we detected a TGF-β time-course-dependent increase of Smad3/N-CoR occupancy at the REGγ promoter in control cells. Conversely, binding of Smad3/N-CoR to the REGγ promoter sharply decreased in p53-R175H-expressing cells. Interestingly, mutant p53 recruited coactivator p300 with increasing strength to the REGγ promoter with TGF-β treatment ( Fig. 5j ). We also obtained similar results in MDA-MB-231 breast cancer cells ( Fig. 5k ). Consistent with previous report that mutant p53 attenuates the TGF-β pathway, we also found reduced phosphorylation of R-smad ( Supplementary Fig. S6a ). Taken together, these data demonstrate that mutant p53, but not p53, is capable of interrupting TGF-β-induced recruitment of Smad complexes to the REGγ promoter by attenuating the DNA-binding capacity of Smad3/4 complex to the corresponding SBE. Furthermore, the switch between the recruitment of N-CoR, which promotes histone deacetylation, and that of p300, which should result in increased histone acetylation, provides additional explanation for the transcriptional activation of REGγ in mutant p53 harbouring cells in response to TGF-β. p53 and TGF-β regulate the 20S proteasome pathway via REGγ To understand whether enhanced REGγ level correlates with its ability to activate proteasome activity, we measured trypsin-like REGγ–20S proteasome activity in multiple human cancer cell lines. To test the effect of p53 on the 20S proteasome activity, we treated A549 cells with ETO and observed that ETO treatment decreased proteasome activity in control cell lines (A549.SHN) but not in REGγ-depleted cell lines (A459.SHR; Fig. 6a and Supplementary Fig. S7a ), suggesting that p53 can inhibit the 20S proteasome pathway via REGγ. Furthermore, we compared isogenic HCT116p53+/+ and HCT116p53−/− cells, and observed that the 20S proteasome activity was much higher in p53−/− cells ( Fig. 6b and Supplementary Fig. S7b ), indicating that p53 can regulate the 20S proteasome pathway. Next, we stimulated A549 cells with TGF-β and found that TGF-β also repressed the 20S proteasome activity in control cells, but not in REGγ-deficient cells ( Fig. 6c ). Intriguingly, mutant p53 was able to enhance the proteasome activity ( Fig. 6d ). Moreover, we detected lower proteasome activity in REGγ knockdown cell lines (ARO.SHR) in the presence of mutant p53, suggesting that mutant p53-induced proteasome activity in ARO cell line depends on REGγ expression ( Fig. 6e and Supplementary Fig. S7c ). Strikingly, mutant p53 was able to attenuate the TGF-β-inhibited proteasome pathway in cancer cells, which explains the mutant p53 GOF ability ( Fig. 6f ). Expectedly, silencing N-CoR enhanced trypsin-like activity, but not in cells with REGγ knockdown cells ( Fig. 6g ). Taken together, these data indicate that p53, TGF-β signalling and mutant p53 regulate the 20S proteasome pathway via REGγ during cancer progression. 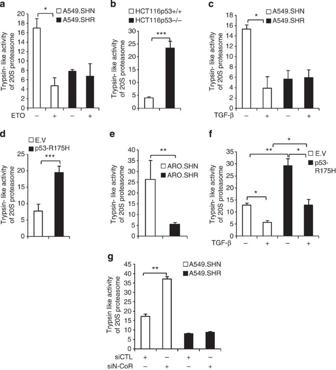Figure 6: Regulation of proteasome pathway by p53/TGF-β via REGγ in cancer cells. (a) p53 suppresses 20S proteasome activity via REGγ. A549 cells were treated with ETO (10 μM) for 24 h and were analysed for trypsin-like activity of 20S proteasome. Data are representative of three biological repeats with mean±s.d. (two-tailed Student’st-test, *P<0.05). (b) p53−/− cells shows higher 20S proteasome activity. HCT116p53+/+ and HCT116p53−/− were compared for analysis of 20S activity. Data are representative of three biological repeats with mean±s.d. (two-tailed Student’st-test, ***P<0.0005). (c) TGF-β inhibits 20S proteasome pathway via REGγ. A549 cells were treated with 5 ng ml−1TGF-β for 24 h and trypsin-like activity of 20S proteasome was determined. Data are representative of three biological repeats with mean±s.d. (two-tailed Student’st-test, *P<0.05). (d) Mutant p53 enhances 20S proteasome pathway via REGγ. H1299 cells stably expressing empty vector (E.V) and p53-R175H were compared for trypsin-like activity of 20S proteasome. Data are representative of three biological repeats with mean±s.d. (two-tailed Student’st-test, ***P<0.0005). (e) Knockdown of REGγ decrease 20S proteasome activity in ARO colon cancer cell lines. Comparison of proteasome activity in control (ARO.SHN) and (ARO.SHR) REGγ-depleted cell lines. Error bars show the mean±s.d. from three technical replicates (two-tailed Student’st-test, **P<0.005). (f) Attenuation of TGF-β inhibited proteasome activity by mutant p53. H1299 cells stably expressing E.V and mutant p53-R175H were left untreated or treated with 5 ng ml−1TGF-β for 24 h and then analysed by proteasome assay. Error bars show the mean±s.d. from three technical replicates (two-tailed Student’st-test, *P<0.05, **P<0.005). (g) Depletion of N-CoR enhances the proteasome pathway. A549 control and knockdown cell lines were transfected with control siRNA or siRNA targeting N-CoR for 72 h and then analysed for proteasome activity. Error bars show the mean±s.d. from three technical replicates (two-tailed Student’st-test, **P<0.005). Figure 6: Regulation of proteasome pathway by p53/TGF-β via REGγ in cancer cells. ( a ) p53 suppresses 20S proteasome activity via REGγ. A549 cells were treated with ETO (10 μM) for 24 h and were analysed for trypsin-like activity of 20S proteasome. Data are representative of three biological repeats with mean±s.d. (two-tailed Student’s t -test, * P <0.05). ( b ) p53−/− cells shows higher 20S proteasome activity. HCT116p53+/+ and HCT116p53−/− were compared for analysis of 20S activity. Data are representative of three biological repeats with mean±s.d. (two-tailed Student’s t -test, *** P <0.0005). ( c ) TGF-β inhibits 20S proteasome pathway via REGγ. A549 cells were treated with 5 ng ml −1 TGF-β for 24 h and trypsin-like activity of 20S proteasome was determined. Data are representative of three biological repeats with mean±s.d. (two-tailed Student’s t -test, * P <0.05). ( d ) Mutant p53 enhances 20S proteasome pathway via REGγ. H1299 cells stably expressing empty vector (E.V) and p53-R175H were compared for trypsin-like activity of 20S proteasome. Data are representative of three biological repeats with mean±s.d. (two-tailed Student’s t -test, *** P <0.0005). ( e ) Knockdown of REGγ decrease 20S proteasome activity in ARO colon cancer cell lines. Comparison of proteasome activity in control (ARO.SHN) and (ARO.SHR) REGγ-depleted cell lines. Error bars show the mean±s.d. from three technical replicates (two-tailed Student’s t -test, ** P <0.005). ( f ) Attenuation of TGF-β inhibited proteasome activity by mutant p53. H1299 cells stably expressing E.V and mutant p53-R175H were left untreated or treated with 5 ng ml −1 TGF-β for 24 h and then analysed by proteasome assay. Error bars show the mean±s.d. from three technical replicates (two-tailed Student’s t -test, * P <0.05, ** P <0.005). ( g ) Depletion of N-CoR enhances the proteasome pathway. A549 control and knockdown cell lines were transfected with control siRNA or siRNA targeting N-CoR for 72 h and then analysed for proteasome activity. Error bars show the mean±s.d. from three technical replicates (two-tailed Student’s t -test, ** P <0.005). Full size image REGγ alters cellular response to p53 and TGF-β signalling Next, we aimed to address the impact of REGγ regulation on p53, TGF-β and mutant p53 cellular activities. We treated the A549 cell lines with anticancer drugs and performed cell proliferation assay. We observed that REGγ knockdown cell lines showed less resistance to ETO and Adriamycin treatment as compared with control cells ( Fig. 7a and Supplementary Fig. S8 ). Thus, depletion of REGγ sensitizes cells to genotoxic insults. Furthermore, we measured apoptotic levels by poly (ADP-ribose) polymerase cleavage (an apoptotic marker). We detected significantly more apoptosis in A549 cells than in ARO cells with stable REGγ knockdown ( Fig. 7b ). Next, we treated A549 cell lines with TGF-β and observed that REGγ-depleted cells were more sensitive to TGF-β treatment and were less proliferative in comparison with control cells ( Fig. 7c ). 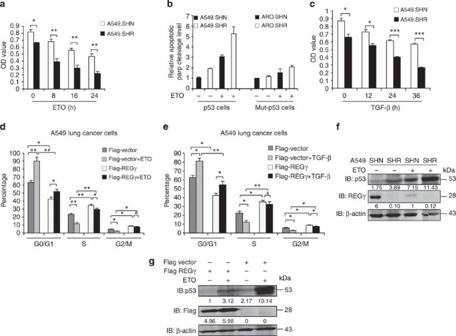Figure 7: REGγ affects p53 and TGF-β signalling cellular response in cancer cells. (a) Knockdown of REGγ decrease drug resistance in A549 lung cancer cells. A549 cells were treated with ETO for indicated time points and then analysed by MTT assay. Error bars show the mean±s.d. from three technical replicates (two-tailed Student’st-test, *P<0.05, **P<0.005). (b) Quantitative comparison for apoptotic level from three independent western blotting experiments. Data show the mean±s.d. from three technical replicates. (c) Knockdown of REGγ restores the tumour suppressor ability of TGF-β. A549 cells were treated with 5 ng ml−1TGF-β at indicated time points, and then MTT assay were performed to check the cell proliferation. Data show the mean±s.d. from three technical replicates (two-tailed Student’st-test, *P<0.05, ***P<0.0005). (d) Overexpression of REGγ enhances cell cycle progression in A459 cells. Flag-REGγ expression plasmid was transfected into A549 parental cells for 24 h, and then left untreated or treated with ETO (10 μmol) for 24 h and analysed by fluorescence-activated cell sorting (FACS) analysis. Data show the mean±s.d. from three technical replicates (two-tailed Student’st-test, **P<0.005 and *P<0.05). (e) Flag-REGγ expression plasmid was transfected into A549 parental cells for 24 h and then left untreated or treated with TGF-β 5 ng ml−1for 24 h. Cells were collected and analysed by FACS analysis. Error bars show the mean±s.d. from three technical replicates (two-tailed Student’st-test, **P<0.005 and *P<0.05). (f,g) Manipulation of REGγ and p53 protein levels mutually affects both protein expressions in cancer cells. (f) A549 SHN and SHR cells were left untreated or treated with ETO (10 μmol l−1) for 24 h and were analysed by western blotting. (g) A549 cells were transfected with flag-REGγ for 24 h and then left untreated or treated with ETO (10 μmol l−1) for 24 h, and were analysed by western blotting. Figure 7: REGγ affects p53 and TGF-β signalling cellular response in cancer cells. ( a ) Knockdown of REGγ decrease drug resistance in A549 lung cancer cells. A549 cells were treated with ETO for indicated time points and then analysed by MTT assay. Error bars show the mean±s.d. from three technical replicates (two-tailed Student’s t -test, * P <0.05, ** P <0.005). ( b ) Quantitative comparison for apoptotic level from three independent western blotting experiments. Data show the mean±s.d. from three technical replicates. ( c ) Knockdown of REGγ restores the tumour suppressor ability of TGF-β. A549 cells were treated with 5 ng ml −1 TGF-β at indicated time points, and then MTT assay were performed to check the cell proliferation. Data show the mean±s.d. from three technical replicates (two-tailed Student’s t -test, * P <0.05, *** P <0.0005). ( d ) Overexpression of REGγ enhances cell cycle progression in A459 cells. Flag-REGγ expression plasmid was transfected into A549 parental cells for 24 h, and then left untreated or treated with ETO (10 μmol) for 24 h and analysed by fluorescence-activated cell sorting (FACS) analysis. Data show the mean±s.d. from three technical replicates (two-tailed Student’s t -test, ** P <0.005 and * P <0.05). ( e ) Flag-REGγ expression plasmid was transfected into A549 parental cells for 24 h and then left untreated or treated with TGF-β 5 ng ml −1 for 24 h. Cells were collected and analysed by FACS analysis. Error bars show the mean±s.d. from three technical replicates (two-tailed Student’s t -test, ** P <0.005 and * P <0.05). ( f , g ) Manipulation of REGγ and p53 protein levels mutually affects both protein expressions in cancer cells. ( f ) A549 SHN and SHR cells were left untreated or treated with ETO (10 μmol l −1 ) for 24 h and were analysed by western blotting. ( g ) A549 cells were transfected with flag-REGγ for 24 h and then left untreated or treated with ETO (10 μmol l −1 ) for 24 h, and were analysed by western blotting. Full size image Moreover, overexpression of REGγ attenuated the effect of ETO and TGF-β on cell cycle progression, and enhanced S and G2/M phase to accelerate DNA synthesis ( Fig. 7d,e and Supplementary Fig. S7e ). Strikingly, REGγ decreased p53 protein expression in the presence or absence of ETO, whereas REGγ knockdown further enhanced p53 protein levels in ETO-treated cell lines ( Fig. 7f,g ), reflecting a regulation of cell cycle progression in a p53-dependent manner. In conclusion, these data show that REGγ depletion decreases drug resistance and sensitizes the cancer cells to chemotherapeutic agents. In addition, overexpression of REGγ affects the tumour suppressive activities of p53 and TGF-β signalling in cancer cells to enhance cancer progression. Knockdown of REGγ arrests growth and cell cycle progression Next, we sought to examine the role of REGγ on cellular growth and cell cycle transition. To this end, we performed MTT (3-(4,5-dimethylthiazol-2-yl)-2,5-diphenyltetrazolium bromide) assay in HCT116p53+/+ and HCT116p53−/− cell lines, in which REGγ was stably knocked down. Intriguingly, we found that in comparison with REGγ-positive HCT116p53+/+ cell line, REGγ-expressing HCT116p53−/− cells (SHN) had markedly enhanced cell proliferation. In contrast, REGγ knockdown (SHR) cells showed reduced proliferation in both HCT116p53+/+ and HCT116p53−/− cell lines ( Fig. 8a ), suggesting that REGγ can further enhance cell proliferation in the absence of p53. Intriguingly, REGγ knockdown led to inhibition of cell proliferation in ARO ( Fig. 8b ) and A549 ( Fig. 8c ) cell lines, suggesting that REGγ promotes cell viability. Next, we assessed the proliferative role of REGγ and mutant p53 in breast cancer cell lines. Importantly, knockdown of REGγ and mutant p53 independently decreased cell growth ( Fig. 8d and Supplementary Figs S7d and S9 ). Strikingly, cosilencing of mutant p53 and REGγ further inhibited cell proliferation in breast cancer cell lines ( Fig. 8d ). These data indicate that REGγ has an important role in cell proliferation of these cancer cell lines in response to p53 signalling. 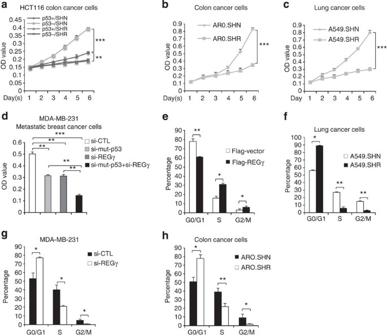Figure 8: Depletion of REGγ inhibits proliferation and cell cycle transition in cancer cells. (a) Isogenic HCT116p53+/+ and HCT116p53−/− cells lines, either expressing REGγ (SHN) or REGγ depleted (SHR) were cultured in 96-well plates for indicated days and were analysed by MTT assay. Error bars show the mean±s.d. from three technical replicates (two-way analysis of variance (ANOVA), ***P<0.0005, **P<0.005). (b) MTT assay; cell proliferation ability was inhibited in ARO REGγ-depleted cells (ARO.SHR). Error bars show the mean±s.d. from three technical replicates (two-way ANOVA, ***P<0.0005). (c) MTT assay; cell proliferation ability was inhibited in A549 REGγ-depleted cells (A549.SHR). Data are representative of three technical repeats with mean±s.d. (two-way ANOVA, ***P<0.0005). (d) MDA-MB-231 cells were transfected with siREGγ (20 nM) and si-mutant p53, either independently or in combination for 72 h, and analysed by MTT assay. Error bars show the mean±s.d. from three technical replicates (two-tailed Student’st-test, ***P<0.0005, **P<0.005). (e) Overexpression of REGγ induces cell cycle transition. Flag-REGγ was transfected into A459 cells for 24 h and then analysed by fluorescence-activated cell sorting (FACS) analysis. Data are representative of three biological replicates with mean±s.d. (two-tailed Student’st-test, *P<0.05, **P<0.005). (f–h) FACS analysis; cell cycle progression was inhibited in (f) A549.SHR-, (g) MDA-MB-231 siREGγ- and (h) AR0.SHR-depleted cells but not in control cell lines. Data are representative of three biological repeats with mean±s.d. (two-tailed Student’st-test, *P<0.05, **P<0.005). Figure 8: Depletion of REGγ inhibits proliferation and cell cycle transition in cancer cells. ( a ) Isogenic HCT116p53+/+ and HCT116p53−/− cells lines, either expressing REGγ (SHN) or REGγ depleted (SHR) were cultured in 96-well plates for indicated days and were analysed by MTT assay. Error bars show the mean±s.d. from three technical replicates (two-way analysis of variance (ANOVA), *** P <0.0005, ** P <0.005). ( b ) MTT assay; cell proliferation ability was inhibited in ARO REGγ-depleted cells (ARO.SHR). Error bars show the mean±s.d. from three technical replicates (two-way ANOVA, *** P <0.0005). ( c ) MTT assay; cell proliferation ability was inhibited in A549 REGγ-depleted cells (A549.SHR). Data are representative of three technical repeats with mean±s.d. (two-way ANOVA, *** P <0.0005). ( d ) MDA-MB-231 cells were transfected with siREGγ (20 nM) and si-mutant p53, either independently or in combination for 72 h, and analysed by MTT assay. Error bars show the mean±s.d. from three technical replicates (two-tailed Student’s t -test, *** P <0.0005, ** P <0.005). ( e ) Overexpression of REGγ induces cell cycle transition. Flag-REGγ was transfected into A459 cells for 24 h and then analysed by fluorescence-activated cell sorting (FACS) analysis. Data are representative of three biological replicates with mean±s.d. (two-tailed Student’s t -test, * P <0.05, ** P <0.005). ( f – h ) FACS analysis; cell cycle progression was inhibited in ( f ) A549.SHR-, ( g ) MDA-MB-231 siREGγ- and ( h ) AR0.SHR-depleted cells but not in control cell lines. Data are representative of three biological repeats with mean±s.d. (two-tailed Student’s t -test, * P <0.05, ** P <0.005). Full size image Next, we aimed to examine the effect of REGγ on cell cycle progression in cancer cell lines. Fluorescence-activated cell sorting analyses showed that overexpression of REGγ enhanced the S (DNA synthesis) and G2/M (mitotic) phase ( Fig. 8e ). Conversely, depletion of REGγ attenuated transition of G0/G1 cells to S and G2/M phases, which are important for cell growth ( Fig. 8f–h ). These data indicate that REGγ promotes cell growth via enhancing DNA synthesis in cancer cells. REGγ expression correlates with mutant p53 in cancer tissues Next, we examined REGγ expression in several human cancer cell lines. In contrast to p53-expressing cancer cell lines, we observed higher expression of REGγ in mutant p53-expressing cells ( Fig. 9a , left panel). Importantly, western blot analysis also showed higher level of REGγ in Smad4-null cells. However, cancer cell lines expressing Smad4 had reduced level of REGγ ( Fig. 9a , right panel). We observed similar results by analysing REGγ transcript in these cancer cell lines ( Fig. 9b,c ). 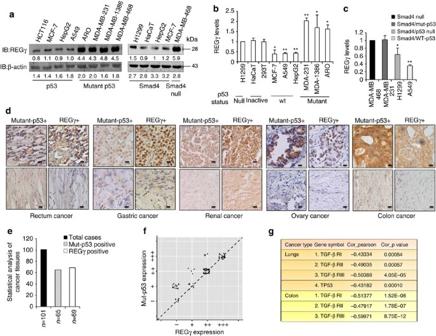Figure 9: REGγ shows a positive correlation with mutant p53 in multiple cancer tissues and cell lines. (a) Western blot analyses of cellular REGγ protein levels in p53- and mutant p53-expressing cancer cells, which is correlated with the p53 status (left panel). Smad4-null cancer cells show more REGγ protein levels in comparison with Smad4-containing cells (right panel). (b) Quantitative RT–PCR analyses of cellular REGγ mRNA levels in four different groups of cancer cells, which are correlated with the p53 status. Error bars show the mean±s.d. from three technical replicates (two-tailed Student’st-test, *P<0.05, **P<0.005). (c) Total RNA was extracted from each of the four different cancer cell lines containing Smad4-null and Smad4-expressing cells. RT–PCR analyses were performed to measure the REGγ mRNA levels. Error bars show the mean±s.d. from three technical replicates (two-tailed Student’st-test, *P<0.05, **P<0.005). (d) Mutant p53 positively correlates with the REGγ. IHC analysis of the multiple cancer tissues, which express different groups of mutant p53 proteins, displayed positive correlation with the REGγ overexpression. Scale bars, 50 μm (shown on × 40 images). (e) Statistical analysis of REGγ and mutant p53-positive cancer tissues. (f) Scatter plot for REGγ and mut-p53 correlation in the same sets of tumours. The scores were put into the plot using the Bland–Altman plot standard method. (g) Bioinformatics analysis of lung and colon cancers, in which overexpression of REGγ negatively correlated with the p53 pathway and TGF-β receptors expression. Pearson’s correlation coefficient was used as a measure of correlation between REGγ and its potentially related genes. Pearson’s correlation analysis was conducted using ‘R programme’ on data set with significant overexpression of REGγ. Figure 9: REGγ shows a positive correlation with mutant p53 in multiple cancer tissues and cell lines. ( a ) Western blot analyses of cellular REGγ protein levels in p53- and mutant p53-expressing cancer cells, which is correlated with the p53 status (left panel). Smad4-null cancer cells show more REGγ protein levels in comparison with Smad4-containing cells (right panel). ( b ) Quantitative RT–PCR analyses of cellular REGγ mRNA levels in four different groups of cancer cells, which are correlated with the p53 status. Error bars show the mean±s.d. from three technical replicates (two-tailed Student’s t -test, * P <0.05, ** P <0.005). ( c ) Total RNA was extracted from each of the four different cancer cell lines containing Smad4-null and Smad4-expressing cells. RT–PCR analyses were performed to measure the REGγ mRNA levels. Error bars show the mean±s.d. from three technical replicates (two-tailed Student’s t -test, * P <0.05, ** P <0.005). ( d ) Mutant p53 positively correlates with the REGγ. IHC analysis of the multiple cancer tissues, which express different groups of mutant p53 proteins, displayed positive correlation with the REGγ overexpression. Scale bars, 50 μm (shown on × 40 images). ( e ) Statistical analysis of REGγ and mutant p53-positive cancer tissues. ( f ) Scatter plot for REGγ and mut-p53 correlation in the same sets of tumours. The scores were put into the plot using the Bland–Altman plot standard method. ( g ) Bioinformatics analysis of lung and colon cancers, in which overexpression of REGγ negatively correlated with the p53 pathway and TGF-β receptors expression. Pearson’s correlation coefficient was used as a measure of correlation between REGγ and its potentially related genes. Pearson’s correlation analysis was conducted using ‘R programme’ on data set with significant overexpression of REGγ. Full size image To further understand the biological relevance of our findings discussed above in tumour development, we evaluated the correlation between REGγ and mutant p53 expression by immunohistochemistry (IHC) analysis of 101 human cancer tissues. We detected a higher percentage of REGγ-positive rates in specimens with p53 overexpression compared with p53-negative groups, suggesting a positive correlation of mutant p53 with REGγ ( Fig. 9d ). The statistical analysis between REGγ and mutant p53 is shown in Fig. 9e and Supplementary Fig. S10a . We analysed the correlation between REGγ and mutant p53 from the same sets of tumours by scatter and agreement plots. These plots indicated that these two proteins are highly associated with each other in the same sets as that of the tumours ( Fig. 9f and Supplementary Fig. S10b ). Furthermore, we performed bioinformatic analysis to check the effect of REGγ overexpression on p53/TGF-β signalling pathway using previously collected data sets (GSE10972, GSE4183, GSE8671, GSE10072, GSE4115 and GSE7670) [14] from the Gene Expression Omnibus database ( http://www.ncbi.nlm.nih.gov/geo/ ). Intriguingly, we found that higher expression of REGγ is correlated with a low level of p53, TGF-β RI, TGF-β RII and TGF-β RIII gene expressions ( Fig. 9g ), further implicating regulatory roles of p53/TGF-β in controlling REGγ and cancer development. In this report, we investigated the previously unknown mechanism for regulation of the REGγ–20S proteasome pathway in cancer cells during tumour development. This study indicates differential regulation of REGγ–20S proteasome pathway by p53/TGF-β signalling and mutant p53 proteins via REGγ in tumour cells. Our results provide the first example that anomaly in p53/TGF-β tumour suppressive signalling deregulates REGγ-mediated ubiquitin/ATP-independent proteasome pathway during tumorigenesis ( Fig. 10a ). REGγ has been found to promote degradation of p53 by acting as a coactivator to promote MDM2-mediated p53 ubiquitination. Depletion of REGγ has been shown to lead to increased p53 protein levels in several cancer cell lines. Together with previous findings, the present study provides a previously unknown model, in which an autoregulatory feedback loop exists between p53 and REGγ. We believe that when p53 is elevated to elicit its biological functions, such as apoptosis, the activity of the REGγ–proteasome pathway will be inhibited to avoid p53 degradation and cell proliferative effects. 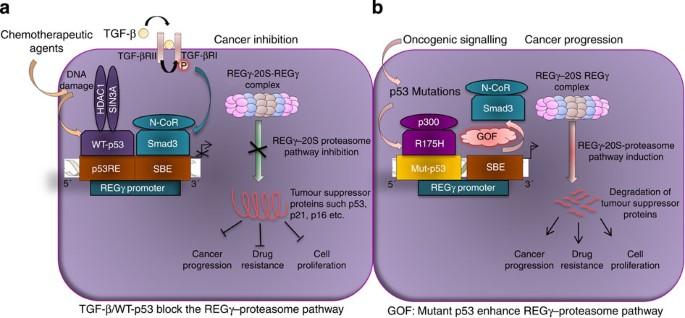Figure 10: Differential regulation of the REGγ–20S proteasome pathway by p53/Smad3 and mutant p53 in cancer cells. A hypothetic model that illustrates (a) both TGF-β and p53 signalling suppress the ubiquitin/ATP-independent REGγ–20Sproteasome pathway via REGγ. Smad3 and p53 proteins negatively regulate REGγ expression through recruitment of its co-repressors. The net output of this mechanism is to prevent the degradation of tumour suppressor proteins and, subsequently, inhibit cancer progression, cell proliferation and decrease drug resistance in cancer cells. (b) Novel GOF of mutant p53: mutant p53 exerts bipartite mechanism to enhance the REGγ–20S proteasome pathway in cancer cells. On one side, mutant p53 binds and recruits p300, a coactivator, and on another side block the recruitment of the Smad3/N-CoR complex formation on REGγ promoter in response to TGF-β. The net gain of this mechanism is to enhance the REGγ–20S proteasome pathway via REGγ in cancer cells to accelerate cancer progression, promote cell proliferation and increase drug resistance during tumour development. Figure 10: Differential regulation of the REGγ–20S proteasome pathway by p53/Smad3 and mutant p53 in cancer cells. A hypothetic model that illustrates ( a ) both TGF-β and p53 signalling suppress the ubiquitin/ATP-independent REGγ–20Sproteasome pathway via REGγ. Smad3 and p53 proteins negatively regulate REGγ expression through recruitment of its co-repressors. The net output of this mechanism is to prevent the degradation of tumour suppressor proteins and, subsequently, inhibit cancer progression, cell proliferation and decrease drug resistance in cancer cells. ( b ) Novel GOF of mutant p53: mutant p53 exerts bipartite mechanism to enhance the REGγ–20S proteasome pathway in cancer cells. On one side, mutant p53 binds and recruits p300, a coactivator, and on another side block the recruitment of the Smad3/N-CoR complex formation on REGγ promoter in response to TGF-β. The net gain of this mechanism is to enhance the REGγ–20S proteasome pathway via REGγ in cancer cells to accelerate cancer progression, promote cell proliferation and increase drug resistance during tumour development. Full size image It is generally believed that the Smad-dependent pathway is involved in TGF-β tumour suppressive functions, whereas activation of Smad-independent pathways is coupled with loss of tumour suppressor function of TGF-β, which is important for its pro-oncogenic effects. Elevated expression of REGγ in both colonic adenoma and invasive cancers suggest that REGγ may have important roles during carcinogenesis. Thus, inhibition of the REGγ–20S proteasome pathway by TGF-β may reduce the risk of cancer development. Combinatorial control of gene expression by p53 and Smad provides a new tier in the regulation of TGF-β gene responses. Our data indicate that neither p53 nor Smads serves as a DNA-binding platform for each other, yet their coexistence greatly augment their binding. Thus, cooperation of p53/TGF-β may fine-tune cytostatic programme in cells by cooperatively regulating the REGγ–20S proteasome pathway. GOF effects of mutant p53 is associated with poor prognosis in cancers. In this study, we show that mutation of p53 enhances REGγ transcription in breast and colon cancer cells. In addition, mutant p53 antagonizes Smad-dependent inhibition of REGγ expression in response to TGF-β by preventing the recruitment of the Smad/N-CoR complex. The accumulated mutant p53 can function as an activator of the REGγ–20S proteasome pathway. Strikingly, mutant p53 recruits p300 on one hand and, on another hand, blocks Smad protein binding. These findings suggest a novel bipartite mechanism by which mutant p53 reprogrammes transcriptional activation of proteasome activator in cancer cells ( Fig. 10b ). Our study highlights the link between p53/TGF-β signalling and the 20S proteasome pathway via REGγ. Our results indicate that both p53 and TGF-β/Smad signalling can inhibit the REGγ–20S proteasome pathway to prevent degradation of important tumour suppressor proteins such as p53/p21/p16. Our data also suggest that REGγ-expressing cells are more resistant to anti-cancer drugs, and knockdown of REGγ decreases chemoresistance in cancer cells. Importantly, we also show that REGγ can attenuate the antiproliferative function of TGF-β/Smad signalling. The opposite behaviour of REGγ in cell proliferation and cell cycle regulation upon silencing p53 or mutant p53 reflect the differential response to distinct p53 signalling and further validate the regulatory mechanisms. Intriguingly, our data also suggest that overexpression of REGγ accelerates DNA synthesis via enhancing S and G2/M phase during tumour development. Strikingly, our IHC analyses show a positive correlation between mutant p53 and REGγ in the rectum, gastric, renal, ovary and colon cancer tissues. Similarly, Smad4-null breast cancer cell lines reveal higher expression of REGγ. Importantly, these analyses indicate that targeting the REGγ–20S proteasome pathway for cancer therapy may be helpful for human tumours having abnormal Smad/p53 proteins status. In addition to this, our bioinformatics data also show that overexpression of REGγ in lung and colon cancer tissues negatively regulates tumour suppressive p53 and TGF-β signalling. Before our studies, no satisfactory mechanism has been proposed for the REGγ–20S proteasome pathway regulation during cancer progression, even though growing evidence suggests that the REGγ–20S proteasome pathway is involved in cancer progression. Plasmids and transfection pcDNA3.1-p53, pcDNA3.1-R175H, pcDNA3.1-R282W, pcDNA3.1-R248W, pcDNA3.1-TA-p63 and pcDNA3.1-TA-p73 were constructed. pRK5-Smad2, pRK5-Smad3 and pRK5-Smad4 were kindly provided by Dr Xin Hua Feng, Baylor College of Medicine. H1299, HeLa, 293T, HaCaT, HCT116 p53−/− and UMSCC-1 cell lines were transfected with Lipofectamine 2000 (Invitrogen) following manufacturer’s protocol. Antibodies The following antibodies were used in western blotting, EMSA assay, ChIP analysis and IHC experiments: Anti-p53 (DO-1, Santa Cruz), anti-p53 (FL393, Cell Signaling Technology), anti-Smad3 (Cell Signaling Technology), anti-Smad4 (Santa Cruz Biotechnology), anti-Smad2 (Santa Cruz Biotechnology), anti-REGγ (Invitrogen), anti-p-smad3 (Cell Signaling Technology), anti-p21(BD Pharmingen), anti-β-actin (Santa Cruz), anti-N-CoR (Abcam), anti-HDAC-1 (Abcam), anti-mSin3a (Abcam), anti-Me-H3K9 (Abcam) and anti-p300 (Santa Cruz). Cell culture and treatments HaCaT, 293T, MCF-7, HepG2, ARO, H1299, A549 were purchased from ATCC. UMSSC-1 (empty vector, p53 and R175H)-expressing cell lines, mouse oral cancer J4708 (p53−/−) and J4705 (p53-R172H) were kind gifts from Dr Carlous Caulin, MD Anderson Cancer Center. HCT116 p53−/− and HCT116 p53+/+ were kind gifts from Dr Bert Vogelstein, John Hopkin University. H1299 cells stably expressing empty vector and p53-R175H were generated. MDA-MB-231 cells were provided by the Tissue Culture Core, Department of Molecular and Cellular Biology, Baylor College of Medicine. MDA-MB-1386 was a kind gift from Dr Jeffery N Myers, MD Anderson Cancer Center. MDA-MB-468 was kindly provided by Dr Xin Hua Feng, Baylor College of Medicine. A549.SHN, A549.SHR, ARO.SHN and ARO.SHR cells were generated. For cell treatments, we used 5 ng ml −1 TGF-β1 (R&D), 10 μmol l −1 Nutlin-3a (Sigma-Aldrich), 5 μg ml −1 cisplatin (Sigma-Aldrich) and (10 μmol) ETO (Sigma-Aldrich). Electrophoretic mobility shift assay EMSA assay was performed with 32 P-radiolabelled probes. Two micrograms of nuclear extract or different concentrations of purified proteins was incubated with 32 P-radiolabelled probes in 20 μl of EMSA assay reaction buffer (2 μg of poly (dI-dC), 20 mM HEPES (pH 7.9), 1 mM MgCl 2 , 40 mM KCl, 0.1 mM EDTA, 1 mM dithiothreitol (DTT) and 12% glycerol). To perform the competition assay, excess of unlabelled competitor’s oligo was added to the EMSA assay reaction mixture. Protein–DNA complexes were resolved in 5% polyacrylamide gels containing 0.5 × Tris-Borate-EDTA (TBE) and exposed to a phoshoimager (Bio-Rad). For the supershift assay, nuclear extracts in the EMSA assay reaction buffer were incubated with different antibodies for 30 min and probes were then added. Probe sequences are described in Supplementary Table S1 . ChIP assay After treatment with TGF-β/Nutlin-3, nuclear proteins were crosslinked to genomic DNA by adding formaldehyde for 10 min directly to the medium to a final concentration of 1%. Crosslinking was stopped by adding glycine to a final concentration of 0.125 M and incubating for 5 min at room temperature on a rocking platform. The medium was removed and the cells were washed twice with ice-cold PBS (140 mM NaCl, 2.7 mM KCl, 1.5 mM KH 2 PO 4 and 8.1 mM Na 2 HPO 4 ·2H 2 O). The cells were collected by scraping in ice-cold PBS supplemented with a protease inhibitor cocktail. After centrifugation, the cell pellets were resuspended in lysis buffer (1% SDS, 10 mM EDTA, protease inhibitors and 50 mM Tris–HCl (pH 8.1)) and the lysates were sonicated to result in DNA fragments of ~200–1,000 bp in length. Cellular debris was removed by centrifugation and the lysates were diluted 1:10 in ChIP dilution buffer (0.01% SDS, 1.1% Triton X-100, 1.2 mM EDTA, 16.7 mM NaCl, protease inhibitors and 16.7 mM Tris–HCl (pH 8.1)). Nonspecific background was removed by incubating the chromatin resuspension with a salmon sperm DNA/protein A agarose slurry for 30 min at 4 °C with agitation. The samples were centrifuged and the recovered chromatin solutions were incubated with 3–5 μg of indicated antibodies overnight at 4 °C with rotation. The immunocomplexes were collected with 60 μl of protein A agarose slurry for 2 h at 4 °C with rotation. The beads were pelleted by centrifugation for 1 min at 4 °C and washed sequentially for 5 min by rotation with 1 ml of the following buffers: low-salt wash buffer (0.1% SDS, 1% Triton X-100, 2 mM EDTA, 150 mM NaCl and 20 mM Tris–HCl (pH 8.1)), high-salt wash buffer (0.1% SDS, 1% Triton X-100, 2 mM EDTA, 500 mM NaCl and 20 mM Tris–HCl (pH 8.1)) and LiCl wash buffer (0.25 mM LiCl, 1% Nonidet P-40, 1% sodium deoxycholate, 1 mM EDTA and 10 mM Tris–HCl (pH 8.1)). Finally, the beads were washed twice with 1 ml TE buffer (1 mM EDTA and 10 mM Tris–HCl (pH 8.0)). The immunocomplexes were then eluted by adding 250 μl elution buffer (1% SDS and 100 mM NaHCO 3 ) and incubated for 15 min at room temperature with rotation. After centrifugation, the supernatant was collected and the crosslinking was reversed by adding NaCl to a final concentration of 200 mM and incubating overnight at 65 °C. The remaining proteins were digested by adding proteinase K (final concentration 40 μg ml −1 ) and incubation for 1 h at 45 °C. The DNA was recovered by phenol/chloroform/isoamyl alcohol (25/24/1) extractions and precipitated with 0.1 volume of 3 M sodium acetate (pH 5.2) and 2 volumes of ethanol using glycogen as a carrier. PCR amplification of the genomic fragments was performed with specific primers flanking putative binding sites on the REGγ promoter. The PCR products were separated by electrophoresis through 2.0% agarose. The primer sequences are described in Supplementary Table S2 . Immunohistochemistry Paraffin-embedded sections (3 μm thick) of different tumours and adjacent normal tissues were used to perform IHC reaction. Tissue sections were deparaffined with xylene and dehydrated with sequential washes of 100, 95 and 70% ethanol. Endogenous peroxidase activity was quenched using 0.3% hydrogen peroxide in methanol for 30 min and then washed in PBS. Antigen retrieval was achieved using a pressure boiler heating in retrieval solution, pH 6, at 125 °C for 4 min, followed by a 20-min cool-down period at room temperature. Slides were then incubated with anti-p53 antibody (1:300) dilutions and anti-REGγ antibody (1:500) dilutions at 4 °C overnight. Next, the slides were rinsed three times in PBS and incubated in biotin-labelled rabbit antirabbit secondary antibodies for 1 h at room temperature. After washing three times with PBS, the staining was performed using 3, 3′-diaminobenzidine. Sections were counterstained with haematoxylin and the staining intensity was evaluated on a scale of 0–2, and was rated as negative (−), weak staining (+), moderate/strong staining (++) and very strong staining (+++). We also compared IHC data between tumours and corresponding adjacent normal tissues by percentage of intensity of staining to estimate the changes of REGγ expression. Production and purification of Smad and p53 fusion proteins Full-length Smad3/Smad4 and p53 proteins fused to glutathione S -transferase were expressed in Escherichia coli and were partially purified by column chromatography using Pharmacia’s protocol. Briefly, bacteria were grown in 2 × YTA medium and induced with 0.1 mM isopropyl-b- D -thiogalactoside. After sonication, glutathione S -transferase fusions were isolated using glutathione Sepharose 4B, washed three times, eluted and then dialysed against PBS supplemented with 2 mM DTT and 0.5 mM phenylmethylsulphonyl fluoride (PMSF). REGγ luciferase reporter constructs DNA fragments containing REGγ genomic sequences were amplified from 293T cell genomic DNA using PCR, and primers were derived from human genomic REGγ and ligated into kpn 1/ xho l sites of the promoterless pGL3-Basic (Promega, Madison, USA) vector and was named as pGL3-REGγ-luc. Different deletion constructs of the REGγ promoter were generated from 1.3 kb REGγ promoter and ligated into kpn 1/ xho l sites of the pGL3-Basic vector. Luciferase assay After transfection and/or treatment, the cells were washed with PBS three times. The cells were then lysed in the luciferase cell culture lysis buffer provided with the Luciferase Assay Kit (Promega). After a brief vortexing, whole-cell lysates were centrifuged in the cold (4 °C) at 13,000 g for 2 min. Supernatant was collected in a fresh tube and 20–30 ml of it was added to the luciferase assay substrate (60–80 ml). Luminescence was measured as relative light units, twice for each lysate, taking the reading of luciferase assay using a LUMIstar OPTIMA (BMG Labtech). Each assay was repeated for three times. Fold repression values were represented as mean of the three experiments. Nuclear extract preparation Cells from 100-mm dishes were washed with PBS and scraped. After another washing, cells were suspended in 2 ml of cold buffer A (20 mM HEPES, pH 7.9, 20 mM NaF, 1 mM Na 3 VO 4 , 1 mM Na 4 P 2 O 7 , 0.13 μM okadaic acid, 1 mM EDTA, 1 mM EGTA, 0.4 mM ammonium molybdate, 1 mM DTT, 0.5 mM PMSF and 1 μg ml −1 each of leupeptin, aprotinin and pepstatin). Cells were allowed to swell on ice for 15 min and then lysed by 30 strokes of a Dounce all-glass homogenizer. Nuclei were pelleted by centrifugation and resuspended in 600 μl of cold buffer C (buffer A, 420 mM NaCl and 20% glycerol). The nucleus membrane was lysed by 15 strokes of a Dounce all-glass homogenizer. The resulting suspension was stirred for 30 min at 4 °C. The clear supernatant was aliquoted and frozen at −80 °C. RNA interference Cells were cultured to 30% confluence. For each well in a 6-well culture dish, 20 nM of Smad3/p53 siRNAs or appropriate negative controls siRNAs was transfected into cells using Lipofectamine 2000 (Invitrogen) following manufacturer’s protocol. Cells were incubated at 37 °C in a CO 2 incubator and, after 6–8 h, 10% serum growth medium was added to the transfection mixture. Cell extracts were assayed by western blotting for Smad3/p53 protein expression at 72 h post transfection, whereas at 48 h after transfection for mRNA expression. The primer sequences are described in Supplementary Table S3 . Reverse transcriptase–PCR Total RNA from cells was isolated using TRIZOL (Invitrogen), following the manufacturer’s protocol. Briefly, 0.5–1 μg of total RNA was reverse-transcribed in a total volume of 25 μl, including 132 units of Moloney–murine–leukemia virus reverse transcriptase, 26.4 units of RNAase inhibitor, 0.6 μg of (dT)15 primer, 2 μM dNTPs and 1 × Moloney–murine–leukemia virus Reverse transcriptase (RT) buffer provided by Promega. Aliquots of the RT products were used for RT–PCR analysis. For semiquantitative RT–PCR analysis, 2 μl of RT products were brought to a volume of 25 μl containing 1.5 mM MgCl 2 , 0.25 mM of each dNTPs, 0.5 μM of both the upstream and downstream PCR primers and 1 × Taq reaction buffer and 1.25 units of Taq DNA polymerase, provided by Promega. PCR products were visualized by electrophoresis on a 2% agarose gel in 0.5 × Tris-borate-EDTA (TBE) buffer after staining with 0.5 μg ml −1 ethidium bromide. For quantitative RT–PCR analysis, 2 μl of reverse-transcribed cDNA was subjected to RT–PCR using mastermix with SYBR-green (Bio-Rad) and the Mx3005P-quantitative RT–PCR system (Stratagene). Each reaction consisted SYBR-green (1:60,000 final concentration), 40 nM of both sense and antisense primers, 2 μl of cDNA and H 2 O to a final volume of 20 μl. Each experiment was performed in duplicates and was repeated three times. Primer sequences are described in Supplementary Table S4 . Preparation of total cell extract and western blot analysis Cells were washed with PBS and treated with an extraction buffer (50 mM Tris–HCl, pH 7.4, 1% Nonidet P-40, 0.25% sodium deoxycholate, 150 mM NaCl and 1 mM EDTA) supplemented with 1 mM PMSF, 1 mM sodium orthovanadate (Na 3 VO 4 ), 0.1 mM DTT, 0.4 μg ml −1 leupeptin/ pepstatin). Cell extract was stored at −20 °C until required. Protein samples were subject to electrophoresis in 10% SDS–PAGE. Separated proteins were electroblotted to nitrocellulose membranes (Bio-Rad), and the blot was blocked for 1 h at room temperature with blocking buffer (0.1% PBS with Tween-20 with 5% fat-free, dried milk powder). The blot was then incubated with primary antibodies, (1:1,000 dilutions) at 4 °C overnight. The blot was washed three times with 0.1% Tris-buffered saline with Tween-20 and incubated with secondary antibodies (mouse, rabbit; 1:5,000 dilution) for 1 h. The blot was washed again three times and exposed to Odyssey LI-COR-scanner. The full-length membranes are shown in Supplementary Figs S11–S18. MTT assay Cell viability was assessed with an MTT assay in replicates. Cells were seeded in 96-well plates at 2.5 × 10 3 cells per well and incubated in 10% fetal bovine serum supplemented with DMEM for 24 h. After that, cells were treated with ETO/TGF-β for indicated time points. Controls received dimethylsulphoxide vehicle at a concentration equal to that in drug-treated cells. Next, drug-containing medium was replaced with 200 μl of 10% fetal bovine serum supplemented with DMEM containing 0.5 mg ml −1 MTT, and cells were incubated in the CO 2 incubator at 37 °C for 2 h and absorbance (490 nm) was measured and analysed. Cell cycle analysis Cell cycle analysis was carried out estimating DNA contents with flow cytometry. Cells were fixed in ice-cold 70% ethanol, incubated overnight at −20 °C and stained with propidium iodide/Triton X-100 containing RNaseA solution for 15 min at 37 °C. Cell cycle analysis was performed using BD CantoII cell analyser. Trypsin-like assay Cells were plated in 96-well plates. After 24 h, cells were treated with TGF-β/ETO for an additional 24 h. Next, 100 μl per well Proteasome-Glo trypsin-like cell-based reagent (catalogue number G8760, Promega) was added and mixed by plate shaking. Luminescence was measured using a luminometer, 15 min after adding the reagent. The Proteasome-Glo cell-based reagents contains a specific luminogenic proteasome substrate in a buffer optimized for cell permeabilization, proteasome activity and luciferase activity. It contains peptide-substrate Z-LRR-aminoluciferin (Z-Leucine-Arginine-Arginine-aminoluciferin) for determination of trypsin-like activity of 20S proteasome. How to cite this article: Ali, A. et al . Differential regulation of the REGγ–proteasome pathway by p53/TGF-β signalling and mutant p53 in cancer cells. Nat. Commun. 4:2667 doi: 10.1038/ncomms3667 (2013).